Backbone rigidity and static presentation of guanidinium groups increases cellular uptake of arginine-rich cell-penetrating peptides In addition to endocytosis-mediated cellular uptake, hydrophilic cell-penetrating peptides are able to traverse biological membranes in a non-endocytic mode termed transduction, resulting in immediate bioavailability. Here we analysed structural requirements for the non-endocytic uptake mode of arginine-rich cell-penetrating peptides, by a combination of live-cell microscopy, molecular dynamics simulations and analytical ultracentrifugation. We demonstrate that the transduction efficiency of arginine-rich peptides increases with higher peptide structural rigidity. Consequently, cyclic arginine-rich cell-penetrating peptides showed enhanced cellular uptake kinetics relative to their linear and more flexible counterpart. We propose that guanidinium groups are forced into maximally distant positions by cyclization. This orientation increases membrane contacts leading to enhanced cell penetration. Beginning with the observation in 1988 that the protein HIV-1 TAT crossed membranes of living cells and altered gene expression [1] , [2] , a variety of so-called protein transduction domains (PTDs) or cell-penetrating peptides (CPPs) have been identified and used to introduce attached cargoes into living cells, organs or animals. For CPPs containing a low number of arginines [3] or carrying large globular cargoes [4] , the mode of cellular uptake is restricted to endocytosis. The well-studied CPPs TAT and artificial oligoarginines belong to the class of arginine-rich CPPs (RRPs). These have, in addition, the option to enter the cell in a non-endocytic mode (hereafter referred to as transduction) with immediate intracellular bioavailability [5] , [6] , if a certain peptide-specific RRP concentration threshold is exceeded. These concentration thresholds depend on the type of RRP as well as on external factors such as the cell line and the extracellular media. Below these concentrations, the main route of RRPs cellular entry seems to be endocytosis. In contrast to pinocytic or endocytic uptake, transduction of RRPs into living cells cannot be prevented by a temperature shift to 4°C (refs 5 , 7 ). Molecular dynamics simulations with TAT solvated in water close to a dioleoloyl phosphatidylcholine lipid bilayer membrane suggested that high concentrations of TAT-peptide can lead to membrane thinning, permitting interactions of arginines with phosphate groups on the opposite leaflet. This event caused the nucleation of a transient, water-filled pore of a size of 3 nm. TAT-molecules diffused along the surface of these pores to the other side of the artificial bilayer [8] . The formation of transient pores on phospholipid bilayers and on cells was later confirmed experimentally [9] . Transient pore formation of TAT is not supported by permanent membrane damage or viability assays in living cells at concentrations slightly above the transduction threshold. This may be attributed to a cellular response towards the peptide incubation, and the ultrashort pore formation may be masked by the activity of a cellular membrane repair response mechanism [10] . RRPs facilitate the delivery of low molecular weight cargoes (for example, peptides up to 30 amino acids, drugs and fluorophores) via the mechanism of transduction and are thus appealing tools to modulate protein function in living cells [11] . Nonetheless, it is still poorly understood which characteristics apart from their arginine content facilitate RRPs to transduce efficiently over the plasma membrane. In this study, we combined live-cell confocal microscopy analysis of cellular uptake of fluorescently labelled peptides, analytical ultracentrifugation and molecular dynamics simulations to define sequence and structural requirements for transduction. In this way, we found that maximal separation of the guanidium groups by cyclization of RRPs enhances their non-endocytic cellular uptake. We propose that this is due to increased membrane contacts facilitated by the rigid cyclic backbone structure. Arginine-rich CPPs rapidly cross plasma membranes To determine the influence of the overall peptide electric charge, the transduction efficiencies of ten different peptides (CPPs, CPP with cargoes and cargoes alone, Supplementary Fig. S1; Supplementary Table S1 ) were evaluated in a live cell fluorescent transduction assay. To strictly score transduced peptides and exclude endocytosed peptides, we analysed the CPPs located in the nucleus. From the panel of CPPs, the well-studied RRPs TAT [12] , [13] and the deca-arginine (R10) peptide [14] , [15] yielded efficiencies of 97% and 98%, respectively. In stark contrast, the CPP PTD 4 (ref. 16 ) could only be found freely diffusing inside cells at a percentage of 0.5% ( Fig. 1a ). All cargoes tested were incapable per se to transduce, although the content of positively charged residues within the sequence increased from Nemo-binding domain [17] without positive charges (c) over the VLC-1 peptide containing four lysines (VLC-1) [18] (b) to p21 consisting of two lysines and five arginines (p21 peptide) [4] (a) ( Supplementary Fig. S1 ). On fusion to the RRP TAT all fusion peptides were able to cross the plasma membrane of living cells in the same manner as TAT alone, albeit with lower transduction frequencies (76–85%), which might reflect the size of the attached cargo or the presence of acidic amino acids within the cargo ( Supplementary Fig. S1 ). 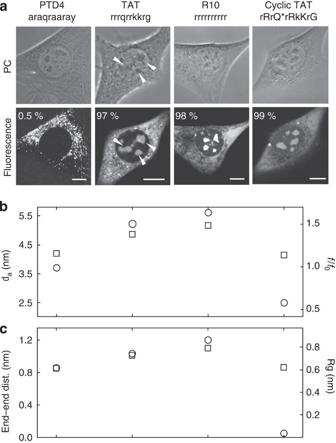Figure 1: Live-cell transduction ability of CPPs and experimental and theoretical shape parameters. (a) The CPPs PTD4, TAT, R10 and cyclic TAT were transduced, or otherwise internalized, into living mouse myoblast cells in the presence of PBS. Representative transmission images of the phase contrast and confocal optical sections of the fluorescent peptides are shown. Scalebars, 10 μm. Arrows indicate the presence of fluorescent peptide inside nucleoli and percentages of the number of transduced cells are given. (b) Results from the sedimentation velocity ultracentrifugation experiments and subsequent analysis:f/f0: frictional ratio (squares), d: diameter, end–end distances (circles). (c) Results of the molecular dynamics simulations: radius of gyration (squares) and end–end distances (circles). Q* results from a decondensation reaction between a glutamic acid and a lysine during cyclization (seeSupplementary Table 1). Figure 1: Live-cell transduction ability of CPPs and experimental and theoretical shape parameters. ( a ) The CPPs PTD4, TAT, R10 and cyclic TAT were transduced, or otherwise internalized, into living mouse myoblast cells in the presence of PBS. Representative transmission images of the phase contrast and confocal optical sections of the fluorescent peptides are shown. Scalebars, 10 μm. Arrows indicate the presence of fluorescent peptide inside nucleoli and percentages of the number of transduced cells are given. ( b ) Results from the sedimentation velocity ultracentrifugation experiments and subsequent analysis: f / f 0 : frictional ratio (squares), d: diameter, end–end distances (circles). ( c ) Results of the molecular dynamics simulations: radius of gyration (squares) and end–end distances (circles). Q* results from a decondensation reaction between a glutamic acid and a lysine during cyclization (see Supplementary Table 1 ). Full size image Arginine-rich CPPs exist as extended and rigid structures A number of studies showed that a minimal number of arginines is required for transduction [6] , [14] , [19] , [20] . Here we further asked whether structural features could explain the high transduction efficiencies of TAT and R10. All peptides from the transduction assay ( Fig. 1a ; Supplementary Fig. S1; Supplementary Table S1 ) were subjected to a sedimentation velocity analytical ultracentrifugation experiment. TAT linked to the fluorophores FITC (fluorescein isothiocyanate), fluorescein and TAMRA (5,6-tetramethyl rhodamine) showed no different intracellular distribution and uptake frequency for either variant ( Supplementary Fig. S2 ), thus ensuring their eligibility for the sedimentation velocity ultracentrifugation experiments. The frictional ratio f / f 0 determined by this analysis allowed the estimation of the gross conformation and dimensions of the peptides ( Fig. 1b ; Supplementary Table S2 ). Frictional ratios around 1 imply sphere-like particles and, with increasing values, the macromolecules can be modelled to more extended and rigid structures. Interestingly, all TAT-containing peptides and R10 exhibited a f / f 0 from 1.29–1.55±0.14 and thus appeared to be extended, whereas the f / f 0 for the non-transducing peptides (without TAT) varied between 1.00–1.16±0.16 hinting towards a more globular shape ( Fig. 1b ; Supplementary Fig. S1; Supplementary Table S2 ). To test whether elongated structure is correlated with positive charge, the f / f 0 was plotted as a function of the charge as well as the number of arginines ( Supplementary Fig. S3 ), showing in fact, an approximately linear correlation between f / f 0 and the number of basic residues. Remarkably, there is among the peptides tested a step-like switch from no transduction to full transduction as the number of basic residues reaches eight including six arginines ( Supplementary Fig. S3 ) [6] . Although the number of charges seems to be important for transduction, it could not be ruled out that the stretched conformation may also have a role. The fact that the p21 peptide exhibits a f / f 0 of 1.40 and thus has an elongated shape as the transducing peptides, but is not able to transduce into living cells ( Supplementary Fig. S1a ), indicates that the extended conformation is not sufficient for transduction. Extended conformation is not essential for transduction To test whether the stretched conformation is a necessary structural property of RRPs, we cyclized the TAT peptide. Analysing the panel of CPPs, implies that, with an increasing number of arginines, the length as well as the frictional ratio increases. There is a sharp drop in both values for the sterically fixed cyclic form of TAT ( Fig. 1b ). To further characterize structural features for the panel of CPPs, probability densities of radius of gyration and end-to-end distances were calculated from molecular dynamics trajectories ( Fig. 1c ). In general, the mean conformational extension increased with the number of arginines, except for the cyclic, sterically constrained TAT peptide, which exhibited a reduced radius of gyration, comparable to the more globular PTD 4 . A comparison between experimentally and theoretically obtained data, revealed the same distribution of values in the graphical space, indicating that experimental and theoretical data were in reasonable agreement ( Fig. 1b,c ). Although, the cyclic TAT has a significantly less stretched conformation than the other CPPs studied, it unexpectedly transduces with frequencies comparable to the other RRPs ( Fig. 1a ). This indicates that extended conformation is neither sufficient nor required for the transduction mode of cellular uptake of CPPs. Cyclic TAT transduces with higher efficiency than linear TAT Surprisingly, the cyclic form of TAT was not only able to translocate into living cells with comparable frequencies as the linear TAT but even exhibited enhanced transduction kinetics ( Fig. 2a,b ; Supplementary Movie 1 ). Although both forms were identically charged, the cyclic TAT variant entered living cells on average 15 min earlier than the linear form and accumulated to higher levels inside the cells (cyclic: 42.0±8.4 min, linear: 69.6±7.1 min). 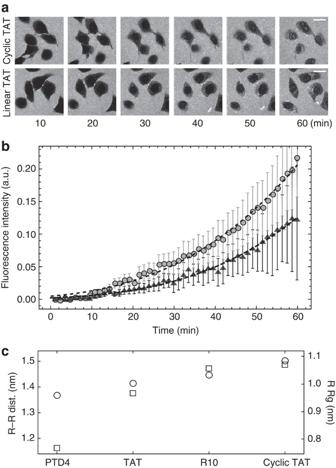Figure 2: Kinetic uptake characteristics of a linear and cyclic form of TAT. (a) Confocal optical sections of timelapse movies (Supplementary Movie 1) show the uptake of fluorescently labelled linear and cyclic TAT in the presence of serum-free medium. Scalebar, 10 μm. (b) Mean fluorescence intensity of fluorescein-labelled linear (triangles) and cyclic (circles) TAT inside the nucleus was monitored over 60 min at a frame rate of one image every 79 s. (c) Radii of gyration (circles) and guanidinium group distances (squares) derived from the molecular dynamics simulations. Figure 2: Kinetic uptake characteristics of a linear and cyclic form of TAT. ( a ) Confocal optical sections of timelapse movies ( Supplementary Movie 1 ) show the uptake of fluorescently labelled linear and cyclic TAT in the presence of serum-free medium. Scalebar, 10 μm. ( b ) Mean fluorescence intensity of fluorescein-labelled linear (triangles) and cyclic (circles) TAT inside the nucleus was monitored over 60 min at a frame rate of one image every 79 s. ( c ) Radii of gyration (circles) and guanidinium group distances (squares) derived from the molecular dynamics simulations. Full size image Guanidinium groups are more distant in cyclic TAT As arginines seem to be the critical ingredient for CPP uptake, we analysed the conformational dynamics of the arginine residues. In Figure 2c ( Supplementary Movies 2 , 3 , 4 , 5 ), it can be seen that although the cyclic peptide has an overall more compact structure, the arginines are more distant than in the linear TAT. As both peptides harbour eight positive charges, the kinetic uptake difference can be attributed to the loss in degrees of freedom in case of the cyclic version, which results in a more rigid presentation of arginine side chains compared with the quite flexible linear variant ( Supplementary Movies 3 and 5 ). As a consequence, the average distance between the guanidinium groups calculated for the cyclic TAT is longer than the one calculated for the other RRPs ( Fig. 2c ), indicating that this is an important parameter for the kinetics of transduction. Larger guanidinium group separation enhances uptake kinetics It has been shown that by increasing the distance between arginine amino acids enhances the uptake of RRPs [25] . This was done by introducing spacers such as glycine amino acids between arginine amino acids. Now, by cyclizing the TAT peptide, we can see that it is possible to increase the distance between the guanidinium groups without performing any mutations of the peptide. If the separation of the guanidium groups is indeed a critical factor for this uptake kinetic difference, then it is expected that this difference should be much pronounced in a peptide composed entirely of arginines. In this case, there is a higher number of guanidinium groups and the arginines are not separated by any other amino acids as in the case of the TAT peptide. To corroborate this kinetical difference, the uptake of cyclic and linear R10 was analysed with the live cell microscopic fluorescence assay. Cyclic R10 transduced several-fold stronger than linear R10, indicated by quicker intranucleolar occurrence and higher intensities over time ( Fig. 3 ). 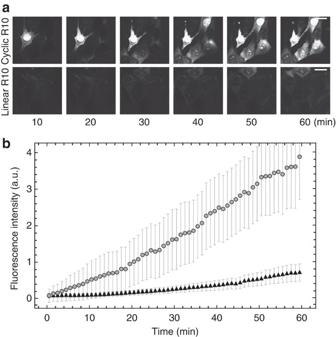Figure 3: Kinetic uptake characteristics of a linear and cyclic form of R10. (a) Confocal optical sections of timelapse movies (Supplementary Movie 6) show the uptake of fluorescently labelled linear and cyclic R10 in the presence of serum-free medium. Scalebar, 10 μm. Because of the much higher cellular uptake of these peptides, the contrast adjustment needed does not allow visualization of the peptide in the extracellular media as in the TAT case (Fig. 2a). (b) Mean fluorescence intensity of fluorescein-labelled linear (triangles) and cyclic (circles) R10 inside the nucleus was monitored over 60 min at a frame rate of one image every 60 s. Figure 3: Kinetic uptake characteristics of a linear and cyclic form of R10. ( a ) Confocal optical sections of timelapse movies ( Supplementary Movie 6 ) show the uptake of fluorescently labelled linear and cyclic R10 in the presence of serum-free medium. Scalebar, 10 μm. Because of the much higher cellular uptake of these peptides, the contrast adjustment needed does not allow visualization of the peptide in the extracellular media as in the TAT case ( Fig. 2a ). ( b ) Mean fluorescence intensity of fluorescein-labelled linear (triangles) and cyclic (circles) R10 inside the nucleus was monitored over 60 min at a frame rate of one image every 60 s. Full size image As predicted, the difference in uptake amount and kinetics between linear and cyclic R10 are far more pronounced than between the TAT counterparts ( Figures 2 and 3 ). We and others have previously reported a concentration-dependent threshold for transduction [4] , [21] and an enrichment of RRPs on the membrane surface [22] , [23] , [24] . On docking to the phospholipids of the plasma membrane, the stabilized outwards presentation of arginines in cyclic TAT might facilitate the formation of RRP assemblies on the cell membranes, initiating transduction earlier than in the case of its linear counterpart. Alternatively, the larger distance between arginines in cyclic TAT may lower the entropic barrier for structures that reach across the membrane, bridging the distance between the polar regions on either side of the lipid bilayer [8] . In linear peptides, it has been observed [25] that enhancing the spacing between arginine residues increases the uptake of RRP suggesting that the spacing between arginine residues is important for uptake. By cyclization of the peptides, as done here, we show that the distance between the guanidinium groups can also be increased without introducing any mutation in the sequence. This also leads to a significant enhancement in the uptake of the TAT peptide narrowing the critical structural aspect to the separation between the guanidium groups. Consequently, this effect is more pronounced in the cyclic R10 peptide that is entirely composed of arginine amino acids. In summary, we show here that the non-endocytic mode of entry by RRPs, termed transduction, depends solely on the number of arginines, and the transduction kinetics of an RRP with a given number of arginines can be enhanced by positional fixation of its guanidinium groups, for example, via backbone cyclization. This restriction in the conformational degrees of freedom can be compared with a state of a statistically reduced number of conformers. This could be achieved also by temperature reduction. Indeed, it has been described that transduction of the linear RRP R9 occurred earlier with decreasing temperature in living cells [7] . Therefore, we propose that a less flexible presentation of arginine side chains distributed over the peptide surface within the cyclic TAT, together with its disc-like appearance, leads to a quicker and more dense occupation of the plasma membrane and thus results in faster transduction kinetics. These features might facilitate the docking process to negatively charged membrane constituents. Consistently, a higher transduction potential of guanidinium groups on a glycoside core that resulted in a semi-rigid conformation has been reported [26] . Altogether, our data suggest that rigidity resulting in an ideal interface for interaction with membrane constituents is more important than structural flexibility [27] to facilitate transduction. We directly show that 'needle'-like structures are not required for transduction and increased distances between the guanidinium groups and structural rigidity kinetically enhances transduction efficiency of arginine-rich CPPs. These findings suggest alternative engineering strategies of novel and more efficient vectors to transport compounds into living cells and organisms. Cells C2C12 mouse myoblasts were seeded at 70% confluency into 8-well microscope observation chambers (ibidi) and the growth medium (Dulbecco's modified Eagle medium; PAA) supplemented with 20% fetal calf serum (Life Technologies) and gentamycin was exchanged against the peptide solutions. Peptides The peptides ( Supplementary Table S1 ) were synthesized using standard Fmoc- and Fboc-chemistry (Peptide Specialty Laboratories BioTez). The cyclization of the cTAT and cR10 peptide was realized between an extra lysine and glutamic acid, which resulted in a TAT-ring with the same overall charge as in the native linear form. Transduction experiments Peptides were diluted to 15 μM final concentration in 200 μl phosphate buffered saline, pH 7.4 (PBS) and incubated with the cells for 60 min at 37°C. Subsequently, the peptide solution was gently exchanged against growth medium. For the timelapses ( Supplementary Movies 1 and 6 ), cells were treated as described above, with the exception that the peptides were diluted in growth medium without fetal calf serum to a final concentration of 20 μM. The UV/VIS absorption spectra for cyclic and linear variants indicated identical peptide concentrations and fluorescent labelling (shown for the linear and cyclic TAT in Supplementary Fig. S4a ). Confocal microscopy and image analysis Confocal microscopy images were acquired with a LSM510 Meta system mounted on an Axiovert 200 M inverted microscope and using a 63x phase contrast planapochromat oil objective NA1.4 (Zeiss). The microscope was equipped with a live-cell incubation chamber maintaining a humidified atmosphere of 5% CO2 and 37°C (Okolab). For all settings, the main beam splitter was HFT UV/488/543/633, and the specific parameters for the single fluorophores were as follows: TAMRA (R) labelled peptides were excited at 543 nm, detected with a 565–615 nm band-pass filter and FITC (F) or fluorescein (Fl) labelled peptides were excited at 488 nm and detected with a 500–530 nm band-pass filter. Phase contrast images were recorded with excitation at 488 nm and detection in the transmission channel. Laser power for observation was 1% at 488 nm, 25 mW and 50% at 543 nm, 1 mW. Settings were adjusted in a way that image pixels were not over or underexposed with the range indicator function in the Zeiss LSM software version 3.2. The macro 'Multi Time Series Rev. 3.2m (ref. 28 ) (Zeiss) was used to record in parallel the uptake of the linear and cyclic variants of TAT in two different wells of the observation chambers. This methodology guaranteed an identical peptide to cell ratio for the measurement, which is crucial for transduction experiments. The uptake movies were generated with the macro 'Concatenate Macro for LSM 3.2 (ref. 28 ) ( Supplementary Movies 1 and 6 ). For the uptake analysis, all extranuclear fluorescence was masked and the increase in fluorescence intensity after peptide application was graphed as average intensity inside whole nuclei. To further correct for small differences, which may arise from heterogeneity of the sample chambers at distinct locations, the histograms taken from the extracellular fluorescence in the movies were compared and the curves obtained for intranuclear fluorescence intensity increase were corrected for this minor differences ( Supplementary Fig. S4b . Furthermore, the graphs were bleach corrected by choosing extracellular ROIs of 80x80 pixels for both peptides. Sedimentation velocity ultracentrifugation analysis The shape parameters of the peptides listed in the Supplementary Table S2 were determined by analytical ultracentrifugation. Molecular mass studies were carried out using an analytical ultracentrifuge XL-A (Beckmann). Minimally 400 μl of the peptides dissolved in 4 mM phosphate buffer, pH 7.45, containing 0.3 M NaCl were centrifuged in standard double sector cells at 50,000 r.p.m. and at 20°C. From the moving boundary, the parameters sedimentation (s) and diffusion (D) coefficients were calculated using the program LAMM [29] . Together with the partial specific volumes, the molecular masses were determined via the Svedberg equation and corresponded in all cases to the expected values for the monomeric peptides. Therefore, as an estimate for the gross conformation, the frictional ratio ( f / f 0 ) was calculated. with , the specific volume of the macromolecule and ρ , the density of the liquid. ( f / f 0 ) is influenced by the two unknown variables shape and hydration. Assuming an average hydration of about 0.3 g bound water per g peptide, a hydration-dependent fraction ( f / f 0 ) hy can be obtained using in which w is the portion of bound water. Division of f / f 0 by the factor ( f / f 0 ) hy yields a shape-dependent frictional ratio ( f / f 0 ) shape , that permits the rough estimation of the molecular dimensions. With the knowledge of the molecular mass M, the dry volume ( V ) can be calculated according to equation 3, with the Avogadro number N A : The dry volumes of the peptides were calculated based on the equation 4 and 5 for the description of sphere-like molecules with the particle radius corresponding to Equation 6 was used for rod-shaped molecules assuming a prolate ellipsoid of revolution with the half-axis a and b (a>b). In case of the cyclic TAT, an oblate ellipsoid of revolution with the half-axis a and b (b>a) was assumed and calculated according to a/b ratios derived from the Oncley-diagram [30] yielded the dry volumes of the peptides. Molecular dynamics simulations For each of the five simulated peptides TAT, cyclic TAT, R10, PTD4, four molecular dynamics simulations over 10 ns were carried out at a temperature of 300 K using GROMACS 3.3.3 (ref. 31 ). The molecules where modelled with the G43a1 force field and immersed in between 2,300 (cyclic TAT) and 7,000 (Nemo-binding domain) water molecules (SPC model). Sodium and chloride counterions were added to achieve overall charge neutrality of the system and physiological ionic strength. To sample a diverse set of conformations, the starting conditions were chosen differently in each simulation by using different random seeds and preparatory high-temperature simulations. Simulations were performed in NVT (number, volume and temperature kept constant) ensemble with periodic boundary conditions and Particle Mesh Ewald treatment of Coulomb interactions. Only the second half of each simulation has been evaluated for the histograms of radius of gyration and end–end distances to avoid biasing by starting conformations. These data are available as Supplementary Movies 2 , 3 , 4 , 5 . How to cite this article: Lättig-Tünnemann, G. et al . Backbone rigidity and static presentation of guanidinium groups increases cellular uptake of arginine-rich cell-penetrating peptides. Nat. Commun. 2:453 doi: 10.1038/ncomms1459 (2011).